Glucocerebrosidase depletion enhances cell-to-cell transmission of α-synuclein Deposition of α-synuclein aggregates occurs widely in the central and peripheral nervous systems in Parkinson’s disease (PD). Although recent evidence has suggested that cell-to-cell transmission of α-synuclein aggregates is associated with the progression of PD, the mechanism by which α-synuclein aggregates spread remains undefined. Here, we show that α-synuclein aggregates are transmitted from cell to cell through a cycle involving uptake of external aggregates, co-aggregation with endogenous α-synuclein and exocytosis of the co-aggregates. Moreover, we find that glucocerebrosidase depletion, which has previously been strongly associated with PD and increased cognitive impairment, promotes propagation of α-synuclein aggregates. These studies define how α-synuclein aggregates spread among neuronal cells and may provide an explanation for how glucocerebrosidase mutations increase the risk of developing PD and other synucleinopathies. Abnormal deposition of α-synuclein aggregates is a pathological feature of Parkinson’s disease (PD) [1] . While a large body of recent studies suggests that transcellular transmission of α-synuclein aggregates is associated with the progression of PD [2] , [3] , [4] , [5] , the mechanisms underlying such transmission are not clearly understood. Particularly urgent issues include whether cell-to-cell transmission of aggregates is seeding-dependent, whether the aggregates disseminates to large cell populations through continuous transmission, and the role of other PD-related genes in this process [6] . Genetic and pathological evidence has suggested that lysosomal impairment is a major contributor in the pathogenesis of Lewy body diseases [7] . The GBA1 gene encodes a lysosomal hydrolase, glucocerebrosidase (GCase), which is deficient in Gaucher disease, the most common lysosomal storage disease. Moreover, mutations in GBA1 are strong genetic risk factors in PD [8] and in dementia with Lewy bodies [9] , although the mechanism by which mutations in GBA1 increase the risk of PD remains unclear. α-Synuclein aggregates that were transferred from cell to cell were transported through the endolysosomal pathway and were degraded in lysosomes [10] , [11] , the finding that prompted us to hypothesize that GBA1 deficiency causes lysosomal dysfunction, thereby increasing the efficiency of aggregate transmission. In the current study, we investigated the mechanism of transmission of α-synuclein aggregates through continuous cell-to-cell transmission and the roles of GCase, a lysosomal enzyme whose mutations represent the most common genetic risk for PD and are implicated in disease severity. Live cell model for aggregate transmission To clarify the mechanism of aggregate propagation by direct observation of cell-to-cell transmission of α-synuclein aggregates, we developed an assay based on bimolecular fluorescence complementation (BiFC), which has been previously successfully applied to assess protein–protein interactions and protein dimerization or oligomerization in living mammalian cells [12] . We produced two stable cell lines expressing α-synuclein fused to either the amino (N) terminus (V1S) or carboxy (C) terminus (SV2) fragment of Venus, a variant of yellow fluorescence protein ( Fig. 1a ). The V1S and SV2 constructs were individually transfected into SH-SY5Y cells, and stable cell lines expressing similar levels of the two α-synuclein fusion proteins were selected ( Fig. 1b ). As anticipated, neither V1S-expressing cells nor SV2-expressing cells fluoresced in individual culture ( Fig. 1d,e ). When the cell lines were cocultured, however, fluorescence resulting from dimerization or oligomerization of the V1S and SV2 fusion proteins [13] during cell-to-cell transfer of α-synuclein was visualized using BiFC ( Fig. 1a,d,e ). Neither the coculture of cells expressing V1S and the C-terminal fragment of Venus (V2) nor those expressing SV2 and the N-terminal fragment of Venus (V1) produced BiFC frourescence ( Supplementary Fig. 1 ), validating the specificity of homotypic interaction between α-synuclein proteins. Since V1S was secreted at a higher level than SV2 ( Fig. 1c ), transfer of α-synuclein during coculture of the cell lines was assumed to primarily involve V1S. 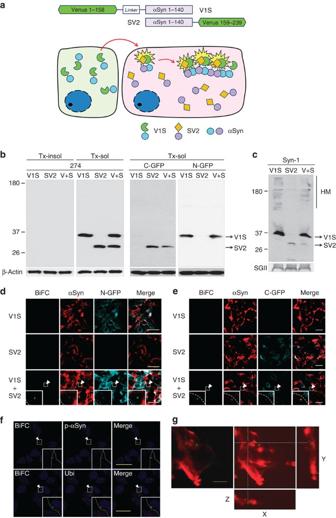Figure 1: Generation of the dual-cell BiFC cell system. (a) Scheme of the dual-cell BiFC system. (b) Western blot analysis of the V1S and SV2 stable cell lines. Primary antibodies used were Ab274 (against human α-synuclein; left panel), anti-GFP C terminus (middle panel) and anti-GFP N terminus (right panel). (c) Western analysis of secreted α-synuclein in the culture media. SgII: secretogranin II, a loading control for secreted proteins. (d,e) Individual cultures and cocultures of V1S and SV2 cell lines were immunostained for α-synuclein and either the N-terminal (d) or C-terminal (e) fragment of Venus. BiFC signal (green) was merged with these immunostains. The boxed regions are magnified in the insets. The dashed lines in the insets represent cell boundaries. Scale bars, 20 μm. (f) BiFC signal (green) merged with phospho-α-synuclein (top panels) and ubiquitin (bottom panels). The boxed regions are magnified in the insets. The dashed lines in the insets represent cell boundaries. Blue: nuclei. Scale bars, 20 μm. (g) A three-dimensional reconstruction of cells containing BiFC fluorescence. Scale bars, 5 μm. Figure 1: Generation of the dual-cell BiFC cell system. ( a ) Scheme of the dual-cell BiFC system. ( b ) Western blot analysis of the V1S and SV2 stable cell lines. Primary antibodies used were Ab274 (against human α-synuclein; left panel), anti-GFP C terminus (middle panel) and anti-GFP N terminus (right panel). ( c ) Western analysis of secreted α-synuclein in the culture media. SgII: secretogranin II, a loading control for secreted proteins. ( d , e ) Individual cultures and cocultures of V1S and SV2 cell lines were immunostained for α-synuclein and either the N-terminal ( d ) or C-terminal ( e ) fragment of Venus. BiFC signal (green) was merged with these immunostains. The boxed regions are magnified in the insets. The dashed lines in the insets represent cell boundaries. Scale bars, 20 μm. ( f ) BiFC signal (green) merged with phospho-α-synuclein (top panels) and ubiquitin (bottom panels). The boxed regions are magnified in the insets. The dashed lines in the insets represent cell boundaries. Blue: nuclei. Scale bars, 20 μm. ( g ) A three-dimensional reconstruction of cells containing BiFC fluorescence. Scale bars, 5 μm. Full size image Immunoflourescence analysis showed that approximately 2–5% of cells contained small fluorescent inclusion bodies positive for α-synuclein and the N and C termini of Venus ( Fig. 1d,e ), phospho-α-synuclein (Ser129) and ubiquitin ( Fig. 1f ). These characteristics are similar to the Lewy bodies and pathogenic inclusions observed in transgenic models [14] , [15] , [16] . Three-dimensional reconstruction of z-stack images indicated that the fluorescent inclusions were intracellular structures ( Fig. 1g ). These results collectively demonstrated the cell-to-cell transfer and co-aggregation of the transferred α-synuclein with resident α-synuclein in the recipient cells, supporting the ‘seeding’ hypothesis of aggregate propagation [3] . Assessed by western analysis, the majority of intracellular α-synuclein in V1S and SV2 cells was Triton X-100 soluble and monomeric ( Fig. 1b ). However, the cell culture media contained the aggregates of α-synuclein ( Fig. 1c ), suggesting the aggregates were preferentially secreted from cells. This is consistent with our previous findings reported by Kim et al . [17] and Jang et al . [18] To further validate the presence of aggregates in the culture media, we performed size-exclusion chromatography using the total culture medium (V1S CM) and the culture medium passed through a 100 kDa cutoff filter (V1S CM-FT) ( Fig. 2a–c ). Histogram of V1S CM showed distribution of α-synuclein in a wide size ranges from monomer (13 ml) to void volume fractions (8 ml), while that of V1S CM-FT showed only the monomer ( Fig. 2b,c ). This suggests that the V1S CM contained aggregated forms, and 100 kDa cutoff filtration effectively removed the aggregates, leaving only the monomers. To confirm the seeded aggregation in the recipient cells, we treated SV2 cells with either the total V1S CM or V1S CM-FT and analysed BiFC-positive aggregates. Administration of the total V1S CM resulted in BiFC-positive aggregates in SV2 cells, whereas removal of high-molecular weight aggregates from the V1S CM (V1S CM-FT) eliminated the ‘seeding’ ability of the CM ( Fig. 2d,e ). These data strongly suggest that cells release aggregated α-synuclein, and the aggregated forms can seed the aggregation in the recipient cells in our dual-cell BiFC model. 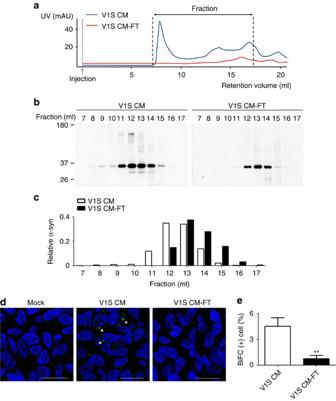Figure 2: α-Synuclein aggregates in V1S CM and their ‘seeding’ effects. (a) Size-exclusion chromatography of V1S CM and V1S CM-FT (the flow-through fraction of 100 kDa cutoff filtration). Blue: V1S CM, Red: V1S CM-FT. (b) Western blotting images of the indicated fractions ina. (c) Quantification of western blot images inb. (d) BiFC fluorescence images in SV2 cells treated with either V1S CM or V1S CM-FT. Scale bars, 20 μm. (e) Percentage of BiFC-positive cells ind. Five hundred cells were analyzed in each of the three independent experiments. **P<0.01 by paired, two-tailed Student’st-test. Figure 2: α-Synuclein aggregates in V1S CM and their ‘seeding’ effects. ( a ) Size-exclusion chromatography of V1S CM and V1S CM-FT (the flow-through fraction of 100 kDa cutoff filtration). Blue: V1S CM, Red: V1S CM-FT. ( b ) Western blotting images of the indicated fractions in a . ( c ) Quantification of western blot images in b . ( d ) BiFC fluorescence images in SV2 cells treated with either V1S CM or V1S CM-FT. Scale bars, 20 μm. ( e ) Percentage of BiFC-positive cells in d . Five hundred cells were analyzed in each of the three independent experiments. ** P <0.01 by paired, two-tailed Student’s t -test. Full size image Continuous cell-to-cell transmission of α-synuclein aggregates To explain pathological aggregate spreading within the central nervous system, cell-to-cell transmission should not be a single discontinuous process. The secondary release of co-aggregated α-synuclein that is produced in the first round of transmission, is absolutely required for spreading of aggregate pathology. To address this problem, we used the dual-cell BiFC system. During continuous subculture of V1S and SV2-expressing cells, if transmission were a single discontinuous event, the percentage of BiFC-positive cells would decrease as passage number increased. Conversely, if the transmission were a continuous event, the percentage of BiFC-positive cells would increase with passage number until reaching a steady state ( Supplementary Fig. 5 ). Coculture of V1S and SV2 cells for several passages (cultured for 48 h for each passage) resulted in a continuous increase in the percentage of BiFC-positive cells ( Fig. 3a,b ). Similarly, BiFC fluorescence in the culture media, representing the secondary secretion of co-aggregates of the ‘seed’ and endogenous α-synuclein, also increased with increasing number of passages ( Fig. 3c ). This was confirmed by increased quantities of oligomers in the media ( Fig. 3d ). We also confirmed that the ratio of BiFC-positive cells between V1S and SV2 cells does not change significantly during the successive subcultures ( Supplementary Fig. 6 ). 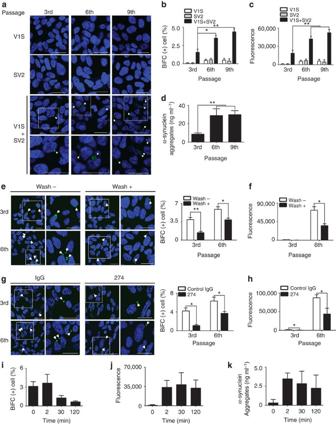Figure 3: Cell-to-cell transmission of α-synuclein aggregates. (a) Subcultures of the dual-cell BiFC system. BiFC-positive inclusions are indicated with arrowheads. Bottom panels are the magnified images of the boxed areas. Scale bars, 20 μm. (b) Quantification of BiFC-positive cells ina.n=4, 1,000 cells per experiment, *P<0.05, **P<0.01 by paired, two-tailed Student’st-test. (c) BiFC fluorescence in the media in the indicated subcultures. **P<0.01 by paired, two-tailed Student’st-test. (d) ELISA specific for α-synuclein multimer in the media of each subculture. **P<0.01 by paired, two-tailed Student’st-test. (e,g) Effects of media wash (e) and Ab274 (g) on percentage of BiFC-positive cells in the indicated subcultures.n=3, 1,000 cells per experiment, *P<0.05, **P<0.01 by paired, two-tailed Student’st-test. (f,h) BiFC fluorescence in the media of the identical cultures ineandg, respectively. (i–k) Conditioned medium of V1S culture was added to SV2 cells for 10 min, and then V1S medium was discarded. The time-dependence of the decay in intracellular BiFC fluorescence (i) was analysed in SV2 cells. Time courses of secondary release of BiFC-positive aggregates (j) and multimeric α-synuclein (k) were analysed in culture media. Figure 3: Cell-to-cell transmission of α-synuclein aggregates. ( a ) Subcultures of the dual-cell BiFC system. BiFC-positive inclusions are indicated with arrowheads. Bottom panels are the magnified images of the boxed areas. Scale bars, 20 μm. ( b ) Quantification of BiFC-positive cells in a . n =4, 1,000 cells per experiment, * P <0.05, ** P <0.01 by paired, two-tailed Student’s t -test. ( c ) BiFC fluorescence in the media in the indicated subcultures. ** P <0.01 by paired, two-tailed Student’s t -test. ( d ) ELISA specific for α-synuclein multimer in the media of each subculture. ** P <0.01 by paired, two-tailed Student’s t -test. ( e , g ) Effects of media wash ( e ) and Ab274 ( g ) on percentage of BiFC-positive cells in the indicated subcultures. n =3, 1,000 cells per experiment, * P <0.05, ** P <0.01 by paired, two-tailed Student’s t -test. ( f , h ) BiFC fluorescence in the media of the identical cultures in e and g , respectively. ( i – k ) Conditioned medium of V1S culture was added to SV2 cells for 10 min, and then V1S medium was discarded. The time-dependence of the decay in intracellular BiFC fluorescence ( i ) was analysed in SV2 cells. Time courses of secondary release of BiFC-positive aggregates ( j ) and multimeric α-synuclein ( k ) were analysed in culture media. Full size image To demonstrate the transfer of seeds through the fluid phase, we next performed media washing and antibody blocking experiments. During the coculture of V1S and SV2 cells, culture media were removed and replaced with the fresh media. When BiFC fluorescence was analysed 1 day after the media replacement, both intracellular and media BiFC signals were decreased ( Fig. 3e,f ), consistent with fluid phase transfer of the seed. Next, we added Ab274, an α-synuclein-specific antibody, to the coculture 1 day before the BiFC analysis, to hijack the secreted α-synuclein, thereby blocking the transfer of this protein. This antibody treatment suppressed BiFC signals in both the cytoplasm and the media ( Fig. 3g,h ). To assess the temporal changes of the seeding and secondary secretion, we conducted a pulse-chase experiment, in which conditioned medium (CM) obtained from the V1S culture was added to the SV2 cells. After a steady state was reached, the V1S CM was washed out and the BiFC signal was analysed in cells and the medium at selected time points. Co-aggregates of V1S and SV2 proteins disappeared rapidly from the cytoplasm after medium washing, whereas the secreted BiFC signal increased reciprocally ( Fig. 3i,j ). Oligomer-specific enzyme-linked immunosorbent assay (ELISA) confirmed the increase in the level of α-synuclein oligomers in the medium ( Fig. 3k ). Together, these results suggest that α-synuclein aggregates are transferred from cell to cell contiguously through a cycle of sequential events, involving intercellular aggregate transfer, seeding of the aggregation of endogenous α-synuclein, and secondary secretion of the seeded aggregates ( Supplementary Fig. 7 ). GBA1 deficiency led to lysosomal dysfunction To assess the role of GBA1 , a strong genetic risk factor for PD, in α-synuclein aggregate transmission, we used a zinc-finger nuclease-based method to establish an SV2 cell line, SV2 GBA1−/− , containing nonsense mutations in both alleles of the GBA1 gene ( Fig. 4a and Supplementary Fig. 8 ). This cell line fails to express GCase 1 ( Fig. 4b ), resulting in greatly reduced total GCase activity ( Fig. 4c ). GCase 2 activity was much lower than the GCase 1 activity, and did not change as a result of GBA1 gene mutation ( Fig. 4d ). As a consequence of depletion of GCase 1, glucosylceramide, a substrate of the enzyme, accumulated in SV2 GBA1−/− cells ( Fig. 4e ). 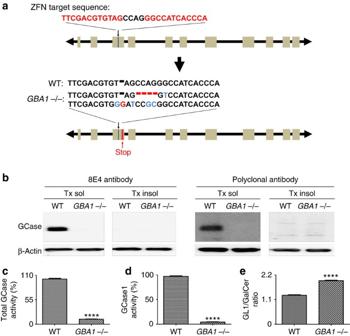Figure 4:GBA1knockout in SV2 cells zinc-finger nucleases. (a) Frame-shift mutations in two alleles of theGBA1gene in SV2 cells. (b) Western blot showing reduced GCase 1 expression in SV2GBA1−/−cells. (c) Reduction of the total GCase activity.n=3, ****P<0.0001 by paired, two-tailed Student’st-test. (d) Specific reduction of GCase 1 activity.n=3, ****P<0.0001 by paired, two-tailed Student’st-test. (e) Increased glucocerebroside (GL1) to galactocerebroside (GalCer) ratio in SV2GBA1−/−cells.n=3, ****P<0.0001 by paired, two-tailed Student’st-test. Figure 4: GBA1 knockout in SV2 cells zinc-finger nucleases. ( a ) Frame-shift mutations in two alleles of the GBA1 gene in SV2 cells. ( b ) Western blot showing reduced GCase 1 expression in SV2 GBA1−/− cells. ( c ) Reduction of the total GCase activity. n =3, **** P <0.0001 by paired, two-tailed Student’s t -test. ( d ) Specific reduction of GCase 1 activity. n =3, **** P <0.0001 by paired, two-tailed Student’s t -test. ( e ) Increased glucocerebroside (GL1) to galactocerebroside (GalCer) ratio in SV2 GBA1−/− cells. n =3, **** P <0.0001 by paired, two-tailed Student’s t -test. Full size image SV2 GBA1−/− cells were characterized by accumulation of lysosomal substrates such as p62 ( Fig. 5a ) and polyubiquitinated proteins ( Fig. 5b ), suggesting lysosomal dysfunction. Consistent with the lysosomal abnormalities, these cells had increased Lysotracker-positive structures ( Fig. 5c ), reduced degradation of ectopically introduced dextran ( Fig. 5d ) and exhibited accumulation of vacuolar structures in the cytoplasm ( Fig. 5e ), all of which clearly demonstrated lysosomal impairment. In addition, we confirmed that GBA1 gene deletion caused lysosomal dysfunction in parental SH-SY5Y cells (data not shown). 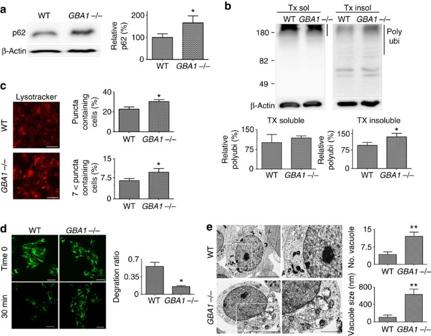Figure 5:GBA1deficiency causes lysosomal dysfunction. (a) Levels of p62 in the Triton-insoluble fractions;n=3, *P<0.05 by paired, two-tailed Student’st-test. (b) Levels of polyubiquitinated proteins. Quantified regions in the blots are indicated by the line on the right;n=4, *P<0.05 by paired, two-tailed Student’st-test. (c) Accumulation of acidic compartments. Five hundred cells were analysed in each of the four independent experiments. Scale bars, 20 μm.n=4, *P<0.05 by paired, two-tailed Student’st-test. (d) Degradation efficiency of internalized dextran-fluorescein isothiocyanate; Scale bars, 20 μm.n=4, 100 cells per experiment, *P<0.05 by paired, two-tailed Student’st-test. (e) Accumulation of endosomal structures. One hundred cells were analyzed. Scale bars, 5 μm (left panels), 2 μm (right panels), **P<0.01 by paired, two-tailed Student’st-test. Figure 5: GBA1 deficiency causes lysosomal dysfunction. ( a ) Levels of p62 in the Triton-insoluble fractions; n =3, * P <0.05 by paired, two-tailed Student’s t -test. ( b ) Levels of polyubiquitinated proteins. Quantified regions in the blots are indicated by the line on the right; n =4, * P <0.05 by paired, two-tailed Student’s t -test. ( c ) Accumulation of acidic compartments. Five hundred cells were analysed in each of the four independent experiments. Scale bars, 20 μm. n =4, * P <0.05 by paired, two-tailed Student’s t -test. ( d ) Degradation efficiency of internalized dextran-fluorescein isothiocyanate; Scale bars, 20 μm. n =4, 100 cells per experiment, * P <0.05 by paired, two-tailed Student’s t -test. ( e ) Accumulation of endosomal structures. One hundred cells were analyzed. Scale bars, 5 μm (left panels), 2 μm (right panels), ** P <0.01 by paired, two-tailed Student’s t -test. Full size image GBA1 deficiency potentiated transmission of α-synuclein We next examined whether GBA1 deletion affects cell-to-cell transmission of α-synuclein. When V1S cells were cocultured with SV2 GBA1−/− cells, the percentage of BiFC-positive cells was significantly increased compared with V1S/SV2 cocultures ( Fig. 6a ). We interpret this to reflect the reduced capacity of SV2 GBA1−/− cells to clear internalized aggregates due to lysosomal impairment ( Fig. 6b ). We then examined the effects of GBA1 gene deletion on contiguous transmission. Coculturing of V1S and SV2 GBA1−/− cells resulted in a significant increase in the number of BiFC-positive cells relative to V1S/SV2 cocultures during several passages ( Fig. 6c,d ). Similarly, levels of α-synuclein oligomers were higher in the media of V1S/SV2 GBA1−/− cocultures than in V1S/SV2 cocultures ( Fig. 6e ; Supplementary Fig. 9 ). Again, the ratio of BiFC-positive cells between V1S and SV2 GBA1−/− did not change significantly during the subculture ( Supplementary Fig. 10 ). Further indicating the role of GCase activity in this process, this phenomenon was reversed by AAV vector-mediated ectopic expression of the wild-type GBA1 gene, but not in that encoding the activity-deficient E235K mutant ( Fig. 6f,g ). 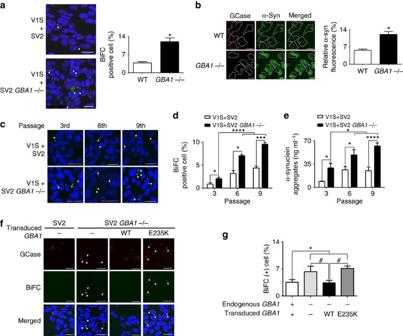Figure 6:GBA1deficiency leads to an increase in cell-to-cell transmission of α-synuclein aggregates. Scale bars, 20 μm. (a) Cell-to-cell α-synuclein transmission in the dual-cell BiFC system. BiFC-positive aggregates are indicated by arrowheads;n=4, 500 cells per experiment, *P<0.05 by paired, two-tailed Student’st-test. (b) Accumulation of ectopically introduced α-synuclein aggregates (sonicated fibrils). Fluorescence was measured in 500 cells in each of the four independent experiments. *P<0.05 by paired, two-tailed Student’st-test. (c) Subcultures of the dual-cell BiFC system. (d) Quantification of BiFC-positive cells shown inc.n=3, 500 cells per each experiment, *P<0.05, ***P<0.005, ****P<0.0001 by paired, two-tailed Student’st-test. (e) Multimeric α-synuclein ELISA analysis of culture media from the indicated subcultures.n=3, *P<0.05, ***P<0.005 by paired, two-tailed Student’st-test. (f,g) Reversal of theGBA1knockout phenotype by expression of wild-typeGBA1, but not the activity-deficient E235KGBA1mutant;n=4, 1,000 cells per each experiment, *P<0.05, #P<0.05 by paired, two-tailed Student’st-test. Figure 6: GBA1 deficiency leads to an increase in cell-to-cell transmission of α-synuclein aggregates. Scale bars, 20 μm. ( a ) Cell-to-cell α-synuclein transmission in the dual-cell BiFC system. BiFC-positive aggregates are indicated by arrowheads; n =4, 500 cells per experiment, * P <0.05 by paired, two-tailed Student’s t -test. ( b ) Accumulation of ectopically introduced α-synuclein aggregates (sonicated fibrils). Fluorescence was measured in 500 cells in each of the four independent experiments. * P <0.05 by paired, two-tailed Student’s t -test. ( c ) Subcultures of the dual-cell BiFC system. ( d ) Quantification of BiFC-positive cells shown in c . n =3, 500 cells per each experiment, * P <0.05, *** P <0.005, **** P <0.0001 by paired, two-tailed Student’s t -test. ( e ) Multimeric α-synuclein ELISA analysis of culture media from the indicated subcultures. n =3, * P <0.05, *** P <0.005 by paired, two-tailed Student’s t -test. ( f , g ) Reversal of the GBA1 knockout phenotype by expression of wild-type GBA1 , but not the activity-deficient E235K GBA1 mutant; n =4, 1,000 cells per each experiment, * P <0.05, # P <0.05 by paired, two-tailed Student’s t -test. Full size image To ensure that the results of the GBA1 gene deletion did not represent ‘off-target’ effects, we next performed RNA interference (RNAi) experiments using AAV vectors. Reduction of GCase 1 expression using two different small hairpin RNAs (shRNAs) was confirmed with western analysis and activity assays ( Supplementary Fig. 11 ). Knockdown of GCase 1 production resulted in a consistent increase in cell-to-cell transfer of α-synuclein. This effect of GCase 1 knockdown was reversed by recovery of GCase 1 production, hence the recovered activity, from ectopic expression of the wild-type GBA1 gene ( Supplementary Fig. 12 ). Collectively, these results show that GBA1 depletion promoted perpetual transmission of α-synuclein aggregates and that ectopic expression of wild-type GBA1 reversed this effect, suggesting that loss of GBA1 function increases α-synuclein aggregate spreading. We have previously shown that transgenic human α-synuclein was transferred from host cells to engrafted cells [10] . To validate the role of GBA1 in vivo , we performed a transplantation experiment in which normal SH-SY5Y cells and GBA1−/− (SH- GBA1−/− ) cells were transplanted into the hippocampus of transgenic mice expressing human α-synuclein, and transfer of α-synuclein from host cells to the grafted cells was analysed. The grafted SH-SY5Y cells do not overexpress α-synuclein, only express small amount of endogenous α-synuclein, which hardly shows up in regular immunological detection protocols ( Fig. 7a–c ). We found that host-derived α-synuclein was deposited at a higher rate in SH- GBA1−/− cells than in normal SH-SY5Y cells ( Fig. 7a–c ). Moreover, co-immunofluorescence analysis showed that SH-SY5Y GBA1−/− cells accumulated host-derived α-synuclein at higher levels than normal SH-SY5Y cells ( Fig. 7d,e ). Note that although SH-SY5Y cells express low levels of endogenous α-synuclein, we failed to detect expression of endogenous α-synuclein in engrafted SH-SY5Y cells ( Fig. 7a–c ). SH-SY5Y cells are human neuroblastoma cells that produce catecholamines, including dopamine. To ensure that our analysis was specific for engrafted cells, we incorporated immunostaining for tyrosine hydroxylase (TH), and found that levels of host-derived α-synuclein were higher in TH-positive engrafted SH-SY5Y GBA1−/− cells than in TH-positive engrafted SH-SY5Y cells ( Fig. 7f,g ). Although there are TH-positive fibres in the hippocampus, there are no TH-positive cells. Thus, TH-positive cells in the hippocampus represent the grafted cells. We also performed a control experiment where differentiated SH-SY5Y cells were tagged with the enhanced green fluorescence protein (eGFP) via lentiviral infection and co-labelled for TH. We found that in in vitro approximately 95% of the eGFP-positive cells were TH-positive. Likewise, about 80% of the grafted SH-SY5Y-eGFP cells in the mouse hippocampus ( n =5) were TH-positive ( Supplementary Fig. 13 ). 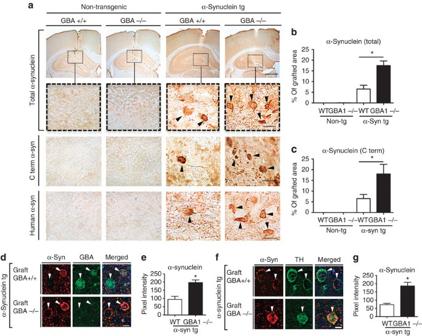Figure 7:GBA1deficiency increases the propagation of α-synuclein pathologyin vivo. (a) Immunohistochemistry of α-synuclein with three different antibodies. Boxed areas in the top panels are magnified in the panels below. Engrafted cells are indicated with arrowheads. Scale bars, top panel, 250 μm; lower panels, 20 μm. (b,c) α-Synuclein immunoreactivities quantified and expressed as a percentage of the grafted area;n=8, *P<0.01 byt-test. (d,e) Co-immunofluorescence analysis of engrafted cells (arrowheads). Pixel intensities of α-synuclein labels measured in 40 cells per animal (n=8). Scale bar, 5 μm. (f,g) Co-immunofluorescence analysis of engrafted cells stained for TH (arrowheads). Pixel intensities of α-synuclein labels measured in 40 cells per animal (n=6). Scale bar, 5 μm. Figure 7: GBA1 deficiency increases the propagation of α-synuclein pathology in vivo . ( a ) Immunohistochemistry of α-synuclein with three different antibodies. Boxed areas in the top panels are magnified in the panels below. Engrafted cells are indicated with arrowheads. Scale bars, top panel, 250 μm; lower panels, 20 μm. ( b , c ) α-Synuclein immunoreactivities quantified and expressed as a percentage of the grafted area; n =8, * P <0.01 by t -test. ( d , e ) Co-immunofluorescence analysis of engrafted cells (arrowheads). Pixel intensities of α-synuclein labels measured in 40 cells per animal ( n =8). Scale bar, 5 μm. ( f , g ) Co-immunofluorescence analysis of engrafted cells stained for TH (arrowheads). Pixel intensities of α-synuclein labels measured in 40 cells per animal ( n =6). Scale bar, 5 μm. Full size image The current study demonstrated that cell-to-cell transmission of α-synuclein aggregates is mediated by a seeding mechanism and that secondary secretion of the resulting seeded aggregates mediates contiguous propagation of α-synuclein aggregates. In addition, the contiguous propagation of aggregates is significantly promoted by lysosomal dysfunction secondary to loss of GBA1 f unction. In PD patients with heterozygous mutations of GBA1 , GCase activities and protein levels were reduced [19] , indicating pathological consequences of GBA1 heteroinsufficiency. Moreover, GBA1 mutation carriers have twice the number of cortical Lewy bodies than those of noncarriers [20] . In addition, heterozygous mutations of GBA1 have been associated with increased risk of cognitive impairment [21] and more rapid disease progression [22] , supporting the hypothesis that the rate of spreading of Lewy pathology determines the rate of clinical progression. The current study provides evidence that α-synuclein transmission is not a single discontinuous event, but a perpetual one. First, continuous subculture of V1S/SV2 coculture showed increased BiFC-positive cell population, instead of its decrease. This observation that there is no dilution effect of BiFC-positive cells as the cell population grows suggests perpetual propagation of α-synuclein aggregates. Second, we found release of BiFC-positive species from V1S/SV2 cocultures, which can only be explained by secondary release of these species after co-aggregation of transferred and resident α-synuclein in the recipient cells. This secondary release of aggregates is a pre-requisite for perpetual propagation of aggregates. Third, ectopic introduction of V1S protein, released from V1S cells, rapidly resulted in BiFC-positive punctates in SV2 cells, and BiFC-positive aggregate species were gradually released from SV2 cells, as cellular BiFC species gradually decreased. These results collectively support the notion that α-synuclein aggregates perpetually propagate through the continuous cycle of exocytosis, endocytosis, seeded aggregation and secondary exocytosis. After several passage of the coculture, the BiFC-positive population reached a steady state, the balance between aggregate production/propagation and degradation as well as cell proliferation rate, which will determine the rate of aggregate dilution. The dilution effect owing to cell proliferation will not be a factor in vivo , since neurons are postmitotic. We suggest that lysosomal degradation is the main force behind the limited increase in BiFC-positive population during successive passages. Increased steady state levels of BiFC-positive cell population with GBA1−/− cells supports this idea. Cell-to-cell transmission we assay with the new dual-cell BiFC system is a relatively infrequent event. We typically observe 2–5% cells with BiFC-positive puncta, though the number varies depending on the culture conditions, such as cell density. The BiFC fluorescence we observe in this system is not an artefact, because either cell line alone rarely shows BiFC signal. Neuroblastoma cells we used in this study produce catecholamines, such as dopamine, which are vulnerable to oxidation. Occasional occurrence of BiFC-positive cells in each cell line is probably due to autofluorescence generated by oxidation of catechols. Although we used extreme caution in handling these cell lines (we only used 2-week to 2-month-old cells), some cells generated this nonspecific background, usually in less than 0.5% of cells. Previous studies showed that α-synuclein can be transferred from neurons to astrocytes [23] and oligodendrocytes [24] . In our dual-cell BiFC system, V1S cells secrete α-synuclein much better than SV2 cells ( Fig. 1 ), so we postulate that V1S cells are the predominant donor cells at least in the initial transfer. In the current study, we intended to investigate the role of GCase 1 in the recipient cells, because the primary goal of the study was to assess the role of lysosomal function in the clearance of transferred α-synuclein and its consequence to aggregates propagation. For this reason, we used SV2 GBA1−/− in this study. However, it will be important to address the role of neuronal GCase 1 activity in neuron-to-glia transmission of α-synuclein in the future studies. Although the current study suggests that loss of GBA1 function has a role in synucleinopathies, this does not necessarily rule out the pathological consequences of gain of GBA1 function mutations. For example, previous studies have associated mutant GBA1 with impaired endoplasmic reticulum-associated degradation [25] and physical interaction between α-synuclein and GCase has been demonstrated under acidic conditions [26] . These studies support a potential role for gain-of-function GBA1 mutations, and stress the point that GBA1 mutations may exert their pathogenic actions via multiple mechanisms. That said, the current study demonstrates that ectopic expression of wild-type GBA1 , but not an activity-deficient GBA1 mutant, reversed the effects of GBA1 deletion on the propagation of α-synuclein aggregates, presenting an attractive therapeutic opportunity for idiopathic PD. These results are in good agreement with previous studies demonstrating amelioration of synucleinopathy lesions in the brains of the GD mouse model (D409V/D409V) by viral-mediated expression of GBA1 (ref. 27 ). Taken together, our work strongly implicates GCase as a disease-modifying therapeutic target, and suggests that restoring the activity of this protein might retard the propagation of Lewy pathology, thereby halting the progression of PD. Materials The following antibodies were used in this study: α-synuclein monoclonal antibody (1:1,500 dilution; BD Biosciences; #610787, San Diego, CA), α-synuclein monoclonal antibody #274 (1:1,500 dilution;), phosphorylated α-synuclein polyclonal antibody (1:100 dilution; Abcam, ab59264; Cambridge, MA), GFP (C terminus) polyclonal antibody (1:100 dilution; IMGENEX, #5127A; San Diego, CA), GFP (N terminus) polyclonal antibody (1:500 dilution; Cell Signaling Technology, #2555; Beverly, MA), GFP (N terminus) monoclonal antibody (1:500 dilution; Abcam, ab127417), GCase monoclonal antibody 8E4 (1:1,000 dilution; from J. Barranger, University of Pittsburgh), GCase polyclonal antibody (1:1,000 dilution; Sigma, G4171; St Louis, MO), p62 monoclonal antibody (1:1,000 dilution; BD Transduction Laboratories, #c2384-0B; Swampscott, MA), ubiquitin polyclonal antibodies (1:1,000 dilution; Dako; Glostrup, Denmark and Chemicon; Temecula, CA), and β-actin monoclonal antibody (1:10,000 dilution; Sigma). Fluorescence dye-conjugated goat anti-rabbit IgG was purchased from Jackson Immunoresearch Laboratories (1:500 dilution; West Grove, PA). The Q tracker 595 cell labelling kit was purchased from Invitrogen (Carlsbad, CA). Construction of stable cell lines To generate stable cell lines, SH-SY5Y human neuroblastoma cells (ATCC CRL-2266; Manassas, VA) were transfected with Venus1-αSyn (V1S) or αSyn-Venus2 (SV2) plasmid (kind gifts from Dr Pamela McLean, Massachusetts General Hospital, Charlestown, MA) using electroporation. Transfected cells were selected with 600 μg ml −1 G418 (Invitrogen) for 2–3 weeks until colonies emerged. The stable cell lines were maintained with 200 μg ml −1 G418. Generation of GBA1 knockout (KO) cell lines SH-SY5Y cells were transfected with plasmids encoding ZFN and a magnetic reporter (ToolGen; Seoul, Korea) using electroporation. After incubation for 48 h, cells were subjected to magnetic separation. After trypsinization, cells were mixed with magnetic bead-conjugated antibody against H-2K k (MACSelect Kk microbeads; Miltenyi Biotech; Germany) and the mixture was applied to a MACS LS column (Miltenyi Biotech). Single cells obtained from the eluates were maintained until the clonal colony was picked from the culture dish. Nonsense mutations in the GBA1 gene were confirmed using DNA sequencing. Cell culture SH-SY5Y human neuroblastoma cell lines were as described previously [28] . Briefly, cells were subcultured at 37 °C in humidified air with 5% CO 2 in Dulbecco’s modified Eagle medium (DMEM) containing 10% fetal bovine serum, 100 units ml −1 penicillin and 100 units ml −1 streptomycin every 2 days. For coculture, V1S and SV2 (or SV2 GBA1−/− ) stable cells (180,000 cells each) were mixed in a coverslip and cultured for 3 days. To determine the continuous transmission of α-synuclein, the mixture of V1S and SV2 (or SV2 GBA1−/− ) cells was subcultured every 2 days (48 h). Growth rates of SV2 and SV2 GBA1−/− were not significantly different during the passage experiment ( Supplementary Fig. 14 ). To determine the effects of media washing on transmission, the V1S/SV2 coculture was washed with DMEM and incubated with fresh growth media the day before assay. To determine the effects of antibodies on the transmission of α-synuclein, 5 μg ml −1 of control IgG or Ab274 was added to V1S/SV2 coculture the day before the assay. Preparation of α-synuclein conditioned media The α-synuclein conditioned media were obtained from 20 dishes of 100-mm dish. When V1S cells are 90% confluent, the medium were replaced with serum-free DMEM after washing three times with DMEM. Cells were incubated at 37 °C for 18 h. Conditioned media (100 ml) were collected from 20 dishes of V1S cells. After centrifugation at 1,000 g for 10 min, supernatant was centrifuged at 10,000 for 20 min to remove the cell debris. The supernatant was concentrated to 200-fold using Amicon 10K MWKO filter (Millipore, Billerica, MA). Size-exclusion chromatography Size-exclusion chromatography was performed using AKTA purifier (GE Healthcare Life Science, Piscataway, NJ). Samples were applied to Superdex 200 HR 10/30 column (GE Healthcare Life Science) equilibrated with phosphate buffer (20 mM sodium phosphate, pH 7.4, 0.15 M NaCl) and eluted at a flow rate of 0.5 ml per minute. GCase activity and glycosphingolipid assay Cellular GCase activity was determined as described previously [27] . Briefly, cells were analysed for GCase activity using 10 mM 4-methylumbelliferyl-β- D -glucoside (Sigma) in buffer containing 1% bovine serum albumin at 37 °C for 1 h. After adding 0.5 volume of 1 M glycine buffer, pH 12.5, cleaved 4-methylumbelliferone was measured using Spectramax Gemini fluorimeter (excitation at 365 nm, emission at 445 nm; Molecular Devices, Sunnyvale, CA). All measurements were done without taurocholate, a detergent that activates the GCase enzymatic activity. GCase2 specific activity was determined in the presence of the GCase 1 inhibitor, conduritol-B-epoxide (100 μM). GCase 1 activity was obtained by subtracting the GCase2 activity levels from the total GCase activity. Cellular GlcCer and GalCer levels were measured by mass spectrometry as previously described [27] . Briefly, organic cellular extracts were injected onto an Atlantis HILIC silica column (Waters Corp.; Milford, MA) for separation of GlcCer and GalCer, which were detected using an AB Sciex API-5000 mass spectrometer. Infection with adeno-associated virus (AAV) vectors After passage, cells were co-infected with Ad-TS129 (3 M.O.I.) and various AAV (5e6 M.O.I.). Cells were incubated at 39 °C for 24 h for activation of the temperature-sensitive helper adenovirus. Several AAV vectors were designed for knockdown of GBA1 ( GFP -miRNA GBA1a and GBA1b ) and a rescue vector expressing a miRNA-resistant GBA1 * ( GBA1 *-miRNA GBA1b ). Quantification of secreted α-synuclein aggregates To measure the level of secreted α-synuclein co-aggregates, culture medium obtained from V1S/SV2 coculture was centrifuged at 10,000 g for 10 min. The supernatant from culture media was transferred to a 96-well black plate (Corning Inc.; Corning, NY) and subjected to fluorometric analysis using a fluorescence microplate reader (SpectraMax Gemini EM;, Molecular Devices, Sunnyvale, CA). The procedure for the ELISA was performed as described previously [29] . Briefly, 1 μg ml −1 of the capture antibody #62 in 50 mM carbonate buffer (pH 9.6) was coated on a 96-well ELISA plate (Maxisorp, Nunc; Rochester, NY) overnight at 4°C. After washing with phosphate-buffered saline (PBS) containing 0.05% Tween 20 (PBST), SuperBlock T20 PBS blocking buffer (Pierce; Rockford, IL) was added for 1 h at room temperature (RT) with shaking. After washing with PBST, α-synuclein aggregates from the standard and culture media were incubated at RT for 2.5 h with shaking. Plates were washed again with PBST, after which 1 μg ml −1 of biotinylated reporter antibody #62 was added and incubated at RT for 1.5 h. After washing with PBST, avidin-conjugated peroxidase (ExtrAvidin; Sigma; St Louis, MO) was added to the plate. The plate was then incubated with 3,3′5,5′-tetramethylbenzidine solution (Sigma). After addition of 2 N H 2 SO 4 , absorbance was measured at 490 nm using a SpectraMax 190 spectrophotometer (Molecular Devices). Preparation of cell extracts After washing with ice-cold PBS, cells were lysed in extraction buffer (1% Triton X-100, 1% (v/v) protease inhibitor cocktail (Sigma) in PBS). Cell lysates were incubated on ice for 10 min and centrifuged at 16,000 g for 10 min. The Triton X-100 insoluble fraction was resuspended in 1X Laemmli sample buffer and sonicated briefly. Western blotting Western blotting was performed as previously described [30] . Images were obtained and quantified using the FUJIFILM Luminescent Image Analyser LAS-3000 and Multi Gauge (v3.0) software (FUJIFILM; Tokyo, Japan). Immunofluorescence staining The procedure for immunofluorescence staining was performed as previously described [30] . Briefly, cells grown on poly- L -Lysine-coated coverslips were fixed in 4% paraformaldehyde in PBS and permeabilized in 0.1% Triton X-100 in PBS. After incubation in blocking solution (5% bovine serum albumin/3% goat serum in PBS), primary antibodies diluted in blocking solution were added to the cells. After washing, cells were incubated with fluorescent dye-conjugated secondary antibodies. Nuclei were stained with TOPRO-3 iodide (Invitrogen). Cells were mounted onto slide glasses in the presence of Prolong Gold Antifade Reagent (Invitrogen). Olympus FV1000 confocal laser scanning microscopy was used for observation of cells. Characterization of lysosomal dysfunction For imaging of the lysotracker-positive compartment, SH-SY5Y cells were stained with 75 nM lysotracker solution in dimethyl sulphoxide (Lysotracker Red DND-99; Invitrogen) diluted in growth media, and incubated for 1 h at 37 °C in a CO 2 incubator. After washing with ice-cold PBS, cells were fixed in a 4% paraformaldehyde (PFA) solution. To determine the degradation ratio of internalized dextran, cells were incubated with 20 μg ml −1 of fluorescein isothiocyanate-labelled dextran (Invitrogen) for 2 h. After washing with DMEM, cells were incubated with fresh growth media for 30 min and fixed with a 4% PFA solution. The fluorescence intensity was measured using Olympus FV1000 software. Electron microscopy Cells were grown in 100-mm dishes and fixed in the Karnovsky’s fixative solution (2% glutaraldehyde, 2% paraformaldehyde, 0.5% CaCl 2 ). After immersing in 1% osmium tetraoxide for 1.5 h, cells were dehydrated with 50, 60, 70, 80, 90, 95 and 100% of absolute ethanol. Cells were infiltrated with propylene oxide and EPON mixture (EPON 812, MNA, DDSA, DMP30) for 10 min before embedding EPON mixture. After embedding, the cells were sectioned with LEICA EM UC-7 Ultra-microtome (Leica Microsystems, Austria), then stained with 6% uranyl acetate and lead citrate. The grids were observed using transmission electron microscopy JEM-1011 (JEOL; Japan) and analysed using Megaview III software (Soft imaging system, Germany). For morphometric analysis, 15 cells were analysed for each experiment. Uptake of extracellular α−synuclein fibrils Cells were incubated with 0.2 μM of sonicated α-synuclein fibrils for 1 day and fixed with 4% PFA. After immunofluorescence staining, the intensity of α-synuclein in a single cell was measured using Olympus FV1000 software. Animals For this study we used heterozygous transgenic mice (Line 61) expressing wild-type human α-synuclein under the control of the mThy1 promoter [31] . These mice were selected since they display extensive neuronal and synaptic accumulation of α-synuclein aggregates throughout the neocortex, limbic system and striato-nigral system, accompanied by motor and nonmotor deficits [32] similar to those observed in patients with PD and dementia with Lewy bodies. Moreover, we have previously shown that α-synuclein in these mice is transmitted from neurons to grafted cells [10] , permitting the evaluation of the effects of GBA1 on transmission. All the procedures for animal experiments were approved by the Institutional Animal Care and Use Committee. Stereotaxic delivery of GBA1−/− cells α-Synuclein transgenic mice and their non-transgenic litter mates ( n =8 per group, 10-month-old, total four groups, 32 mice) received unilateral stereotaxic injections of a 2 μl suspension of wild-type or GBA1−/− cell preparation (1.2 million cells) into the hippocampus as previously described [10] . Mice were anaesthetized and placed on a Koft stereotaxic apparatus. Utilizing an electronic delivery pump system, SH-SY5Y or SH-SY5Y GBA−/− cell preparations were injected using a Hamilton syringe. Coordinates for the hippocampus were as follows: AP −2.0 mm, lateral 1.5 mm, depth 1.3 mm. Mice survived for 4 weeks after the graft injection. Following NIH guidelines for the humane treatment of animals, mice were anaesthetized with chloral hydrate and flush-perfused transcardially with 0.9% saline. Brains were removed and fixed in phosphate-buffered 4% PFA (pH 7.4) at 4 °C for 48 h for neuropathological analysis. Immunocytochemical analysis and confocal microscopy Brains were serially sectioned at 40 μm using a vibratome (Leica; Deerfield, IL, USA). Serial, free-floating, blind-coded vibratome sections from transgenic and non-transgenic mice grafted with WT and SH-SY5Y GBA1−/− cells were immunostained as previously described [33] with antibodies against total α-synuclein (Millipore), α-synuclein C terminus (SYN105 antibody), and human α-synuclein (SYN211). Sections were then incubated with biotin-tagged secondary antibodies and developed with diaminobenzidine. Sections immunolabeled with antibodies against α-synuclein (three from each mouse at 100-μm intervals) were analysed via the dissector method using the Stereo-Investigator System (MBF Bioscience; Williston, VT) and the results were averaged and expressed as the percentage of positive cells in the grafted area. To determine the colocalization between α-synuclein and neuronal markers, double-labelling experiments were performed, as previously described [34] . For this purpose, vibratome sections were immunolabeled using an antibody against human α-synuclein (SYN211) and antibodies against TH (Millipore) and GCase (Abcam, ab55080). The TH- and GCase-immunoreactive grafted cells were detected with fluorescein isothiocyanate-tagged antibodies (1:75; Vector; Burlingame, CA), while α-synuclein was detected with Tyramide Red (NEN Life Sciences). All sections were processed simultaneously under the same conditions, and experiments were performed in duplicate to assess the reproducibility of results. Sections were imaged with a Zeiss 63X (N.A. 1.4) objective on an Axiovert 35 microscope (Zeiss) with an attached MRC1024 laser scanning confocal microscope (LSCM) system (BioRad) [34] . Series of paired optical sections were analysed with ImageJ colocalization colour map software to determine the α-synuclein pixel intensity associated with WT and GBA1−/− cells. An average of 20 digital images was analysed per mouse. Each digital image contained an average of four cells. Values in the figures are expressed as means±s.e.m. Statistical analysis Values shown in the figures are presented as mean±s.e.m. To determine the statistical significance, P values were calculated by means of paired, two-tailed Student’s t -tests using GraphPad InStat version 3.05 software. How to cite this article: Bae, E.-J. et al . Glucocerebrosidase depletion enhances cell-to-cell transmission of α-synuclein. Nat. Commun. 5:4755 doi: 10.1038/ncomms5755 (2014).